Chitosan confinement enhances hydrogen photogeneration from a mimic of the diiron subsite of [FeFe]-hydrogenase Nature has created [FeFe]-hydrogenase enzyme as a hydrogen-forming catalyst with a high turnover rate. However, it does not meet the demands of economically usable catalytic agents because of its limited stability and the cost of its production and purification. Synthetic chemistry has allowed the preparation of remarkably close mimics of [FeFe]-hydrogenase but so far failed to reproduce its catalytic activity. Most models of the active site represent mimics of the inorganic cofactor only, and the enzyme-like reaction that proceeds within restricted environments is less well understood. Here we report that chitosan, a natural polysaccharide, improves the efficiency and durability of a typical mimic of the diiron subsite of [FeFe]-hydrogenase for photocatalytic hydrogen evolution. The turnover number of the self-assembling system increases ~4,000-fold compared with the same system in the absence of chitosan. Such significant improvements to the activity and stability of artificial [FeFe]-hydrogenase-like systems have, to our knowledge, not been reported to date. Enzymes may bind substrates through multiple interactions in elaborate pockets to direct a specific reaction pathway under mild conditions [1] , [2] , [3] , [4] . [FeFe]-hydrogenase ([FeFe]-H 2 ase) [5] , [6] , a natural enzyme for hydrogen (H 2 ) evolution, is deeply embedded within the protein matrix to enable the reversible reduction of protons to H 2 with low overpotential and high turnover frequencies (TOF 6,000–9,000 s −1 per catalytic site). The high-resolution X-ray crystallographic structures establish that [FeFe]-H 2 ase, isolated from Desulfovibrio desulfuricans [5] and Clostridium pasteurianum [6] , features a butterfly [Fe 2 S 2 ] subunit coordinated by a cysteine-linked [Fe 4 S 4 ] cluster, carbon monoxide and cyanide ligands, and by a dithiolate bridging the two iron centres. The diiron [Fe 2 S 2 ] subunit serves as the catalytic centre for proton reduction, and the [Fe 4 S 4 ] cluster mediates transfer electron to and from the active site of the H-cluster. The astonishing rates of H 2 production from the non-precious diiron catalysts via a group of enzymes under mild conditions can exceed those of platinum. However, the large-scale isolation of the enzyme from natural systems is rather difficult, hence the development of artificial [FeFe]-H 2 ase analogues capable of reproducing the enzymic activity has spurred considerable interest in both the scientific and industrial communities [7] , [8] , [9] , [10] , [11] , [12] , [13] , [14] , [15] , [16] , [17] , [18] , [19] , [20] , [21] , [22] , [23] , [24] , [25] . Over the past decade, a variety of mimics of the diiron subsite of [FeFe]-H 2 ase have been shown to function as catalysts for chemical reduction of protons [26] , [27] , [28] , [29] , [30] , [31] , [32] , [33] . It has been clear that electron transfer, either electrochemical or photochemical, to a mimic of the active site of [FeFe]-H 2 ase is a prerequisite for H 2 evolution [10] , [11] , [12] , [13] , [14] , [22] . From a photochemical point of view, the electron transfer is triggered by the absorption of a photon by a photosensitizer [13] , [14] , [15] , [16] , [17] , [18] , [19] , [20] , [21] , [22] , [23] , [24] , [25] . Since the first attempt by Sun and Åkermark [34] to construct an artificial photocatalytic system for H 2 evolution in 2003, a large number of synthetic model complexes have been pursued to mimic the structure and functionality of the diiron subunit of the natural [FeFe]-H 2 ase H-cluster [35] , [36] , [37] , [38] , [39] , [40] , [41] , [42] , [43] , [44] , [45] , [46] , [47] , [48] , [49] , [50] , [51] . It is encouraging to see that the catalytic efficiency for H 2 evolution from artificial photocatalytic systems using mimics of the diiron subsite of [FeFe]-H 2 ase as catalysts has been increased from null to more than hundreds or thousands of turnover numbers (TON) under different irradiation conditions. In comparison to the efficient diiron active site of [FeFe]-H 2 ase in nature, however, no [FeFe]-H 2 ase mimic has been able to duplicate the high level of reactivity of natural [FeFe]-H 2 ase. Review of the literature indicates that the synthetic mimics of [FeFe]-H 2 ase reported thus far are mainly focused on the inorganic cofactor only, and the enzyme-like reaction that proceeds within restricted environments is to date poorly understood. With this in mind, we initiated the study of a chitosan-confined mimic of the diiron subsite of [FeFe]-H 2 ase for H 2 production. Chitosan is a naturally occurring polysaccharide containing a significant content of primary amines and hydroxyl groups [52] , [53] , [54] . When the amines are protonated by acids, chitosan bears a polycationic character. In view of the chelation and electrostatic interactions, we envision that chitosan may incorporate mimics of the diiron subsite of [FeFe]-H 2 ases intimately, as is the case of [FeFe]-H 2 ase, which is buried deeply within the protein matrix in nature. To avoid side-chain effects, the simplest mimic of the diiron subsite of [FeFe]-H 2 ases, [Fe 2 (CO) 6 (μ-adt)CH 2 C 6 H 5 ] [μ-adt=N(CH 2 S) 2 ] [27] , [37] , is selected as a catalyst ( Fig. 1 ). The 3-mercaptopropionic acid (MPA)-capped CdTe quantum dots (MPA-CdTe QDs), promising for H 2 evolution in combination with a mimic of the diiron subsite of [FeFe]-H 2 ase (ref. 45 ), are used as the photosensitizer. Herein, CdTe QDs are stabilized by MPA and their negatively charged surfaces [55] preferably interact with cationic chitosan. Ascorbic acid (H 2 A) serves as not only a proton source to protonate the amines of chitosan and the catalytic intermediate of photoreduced mimic of the diiron subsite of [FeFe]-H 2 ase but also as a sacrificial electron donor to regenerate MPA-CdTe QDs for photocatalytic H 2 production. Significantly, the self-assembled system that comprises chitosan, [Fe 2 (CO) 6 (μ-adt)CH 2 C 6 H 5 ], MPA-CdTe QDs and H 2 A is capable of producing H 2 with TON of up to (5.28±0.17) × 10 4 and initial TOF of 1.40±0.22 s −1 with respect to [Fe 2 (CO) 6 (μ-adt)CH 2 C 6 H 5 ] catalyst under visible light irradiation ( λ >400 nm). The catalytic stability is enhanced from 8 to 60 h and the catalytic activity is over 4.16 × 10 3 -fold higher than that of the same system without chitosan. The activity and stability are, to the best of our knowledge, the highest to date for light-driven catalytic H 2 evolution from mimics of the diiron subsite of [FeFe]-H 2 ase. 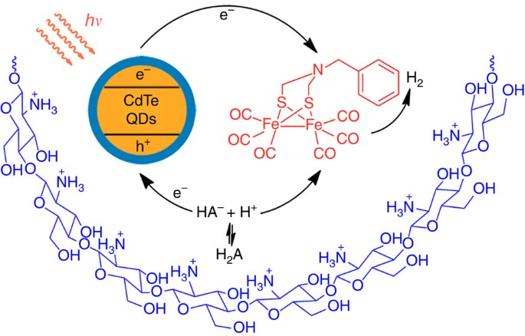Figure 1: Chitosan-confined H2photogeneration. A schematic describing the H2photogeneration of a chitosan-confined mimic of the diiron subsite of [FeFe]-H2ase in the presence of CdTe quantum dots and H2A. Figure 1: Chitosan-confined H 2 photogeneration. A schematic describing the H 2 photogeneration of a chitosan-confined mimic of the diiron subsite of [FeFe]-H 2 ase in the presence of CdTe quantum dots and H 2 A. Full size image The photocatalytic activity of H 2 evolution An initial photocatalytic experiment of [Fe 2 (CO) 6 (μ-adt)CH 2 C 6 H 5 ] catalyst with MPA-CdTe QDs was evaluated in the absence of chitosan. To keep the solubility of [Fe 2 (CO) 6 (μ-adt)CH 2 C 6 H 5 ] catalyst throughout the experiment, we carried out the reaction in a mixture of methanol and water. The anaerobic solution, containing [Fe 2 (CO) 6 (μ-adt)CH 2 C 6 H 5 ] catalyst (1.00 × 10 −5 mol l −1 ), MPA-CdTe QDs (0.86 × 10 −6 mol l −1 ), along with H 2 A (0.10 mol l −1 ), was irradiated by light-emitting diodes ( λ =410 nm) at room temperature, where the best ratio of methanol to water was found to be 1:3 (v-v) ( Supplementary Fig. S1 ). The photoproduct of H 2 was characterized by gas chromatography (GC) analysis with methane as the internal standard. The time course showed that the amount of H 2 increased in the first 4 h and then leveled off, yielding a TON of only 1.74±0.06 based on [Fe 2 (CO) 6 (μ-adt)CH 2 C 6 H 5 ] catalyst ( Fig. 2a , line A). In sharp contrast, the catalytic performance of the same solution was improved significantly in the presence of 1.0 g l −1 of chitosan. Line B in Fig. 2a shows the H 2 production over time from the mixture under visible light irradiation. The amount of H 2 reached 1.27±0.01 ml (TON=569±2) within 10 h of irradiation, and the rate of H 2 evolution was almost linear even after 10 h of irradiation. Control experiments further proved that the components in the system, [Fe 2 (CO) 6 (μ-adt)CH 2 C 6 H 5 ] catalyst, MPA-CdTe QDs, H 2 A, chitosan or light are all essential for efficient H 2 generation. The absence of [Fe 2 (CO) 6 (μ-adt)CH 2 C 6 H 5 ] catalyst led to the rate of H 2 evolution dropping dramatically and no H 2 could be detected when either MPA-CdTe QDs or H 2 A was absent from the reaction system with chitosan ( Supplementary Fig. S2 ). The difference in the catalytic activity (1.74 versus 569) and stability (4 versus 10 h) for the systems with and without chitosan under the same condition implies that chitosan has a key role in the photocatalytic H 2 evolution. 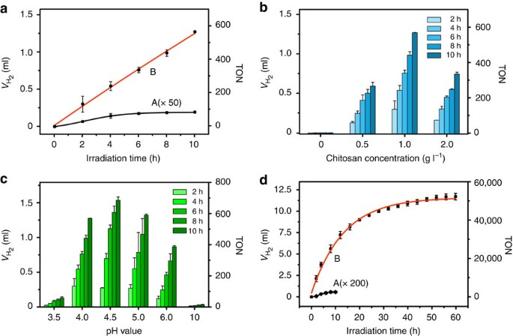Figure 2: H2evolution under visible light irradiation. (a) H2evolution in the absence (A) and presence (B) of chitosan (1.0 g l−1), containing MPA-CdTe QDs (0.86 × 10−6mol l−1), [Fe2(CO)6(μ-adt)CH2C6H5] catalyst (1.00 × 10−5mol l−1) and H2A (0.10 mol l−1) in methanol/water (1:3 v-v); (b) H2evolution as a function of chitosan concentrations, containing MPA-CdTe QDs (0.86 × 10−6mol l−1), [Fe2(CO)6(μ-adt)CH2C6H5] catalyst (1.00 × 10−5mol l−1) and H2A (0.10 mol l−1) in methanol/water (1:3 v-v); (c) H2evolution at various pH values, containing MPA-CdTe QDs (0.86 × 10−6mol l−1), [Fe2(CO)6(μ-adt)CH2C6H5] (1.00 × 10−5mol l−1), H2A (0.10 mol l−1) and chitosan (1.0 g l−1) in methanol/water (1:3 v-v); (d) H2evolution under the optimized conditions in the absence (A) and presence (B) of chitosan, containing MPA-CdTe QDs (1.71 × 10−6mol l−1), [Fe2(CO)6(μ-adt)CH2C6H5] (1.00 × 10−6mol l−1) and H2A (0.20 mol l−1) in methanol/water (1:3 v-v) at pH 4.5. Error bars represent mean±s.d. of parallel experiments. Figure 2: H 2 evolution under visible light irradiation. ( a ) H 2 evolution in the absence (A) and presence (B) of chitosan (1.0 g l −1 ), containing MPA-CdTe QDs (0.86 × 10 −6 mol l −1 ), [Fe 2 (CO) 6 (μ-adt)CH 2 C 6 H 5 ] catalyst (1.00 × 10 −5 mol l −1 ) and H 2 A (0.10 mol l −1 ) in methanol/water (1:3 v-v); ( b ) H 2 evolution as a function of chitosan concentrations, containing MPA-CdTe QDs (0.86 × 10 −6 mol l −1 ), [Fe 2 (CO) 6 (μ-adt)CH 2 C 6 H 5 ] catalyst (1.00 × 10 −5 mol l −1 ) and H 2 A (0.10 mol l −1 ) in methanol/water (1:3 v-v); ( c ) H 2 evolution at various pH values, containing MPA-CdTe QDs (0.86 × 10 −6 mol l −1 ), [Fe 2 (CO) 6 (μ-adt)CH 2 C 6 H 5 ] (1.00 × 10 −5 mol l −1 ), H 2 A (0.10 mol l −1 ) and chitosan (1.0 g l −1 ) in methanol/water (1:3 v-v); ( d ) H 2 evolution under the optimized conditions in the absence (A) and presence (B) of chitosan, containing MPA-CdTe QDs (1.71 × 10 −6 mol l −1 ), [Fe 2 (CO) 6 (μ-adt)CH 2 C 6 H 5 ] (1.00 × 10 −6 mol l −1 ) and H 2 A (0.20 mol l −1 ) in methanol/water (1:3 v-v) at pH 4.5. Error bars represent mean±s.d. of parallel experiments. Full size image Furthermore, the amounts of chitosan together with MPA-CdTe QDs and [Fe 2 (CO) 6 (μ-adt)CH 2 C 6 H 5 ] catalyst were carefully investigated to optimize the reaction. Note that 1.0 g l −1 chitosan is the best concentration to achieve the highest TON of the assembled system for H 2 evolution under a given pH condition ( Fig. 2b ). And the smaller size of MPA-CdTe QDs that is emissive at shorter wavelength gives rise to the higher TON for the photocatalytic H 2 evolution system ( Supplementary Fig. S3 ). The highest TON was obtained in the presence of MPA-CdTe QDs Green (2.8 nm) ( Supplementary Table S1 ). As the conduction band energy of MPA-CdTe QDs Green is over −2.0 V, we could detect a small amount of H 2 from the system without catalyst ( Supplementary Fig. S2 ). Under the same condition, that is, 10 ml methanol/water solution (1:3, v-v) containing chitosan (1.0 g l −1 ), MPA-CdTe QDs (0.86 × 10 −6 mol l −1 ) and H 2 A (0.10 mol l −1 ) at pH 4.0, the amount of H 2 was 6.61±0.48 μl per 10 h in the absence of catalyst. However, the presence of catalyst, [Fe 2 (CO) 6 (μ-adt)CH 2 C 6 H 5 ] (1.00 × 10 −5 mol l −1 ), resulted in H 2 evolution efficiently (1.27±0.01 ml per 10 h). Moreover, the rate of H 2 evolution increased as a function of the concentration of [Fe 2 (CO) 6 (μ-adt)CH 2 C 6 H 5 ] catalyst ( Supplementary Fig. S4 ). When the concentration of the catalyst was higher than 1.00 × 10 −5 mol l −1 , where the ideal concentration of MPA-CdTe QDs was 1.71 × 10 −6 mol l −1 ( Supplementary Fig. S5 ), the rate of H 2 evolution would be no longer linear. In this situation, the highest TON value was achieved at 1.00 × 10 −6 mol l −1 of [Fe 2 (CO) 6 (μ-adt)CH 2 C 6 H 5 ] ( Supplementary Fig. S4 ), the optimal ratio of MPA-CdTe QDs to [Fe 2 (CO) 6 (μ-adt)CH 2 C 6 H 5 ] catalyst is therefore 1.7:1. It was worth noting that the pH value is the most important factor that governs the performance of photocatalytic H 2 evolution. Figure 2c shows pH effect on the H 2 evolution under the same concentrations of [Fe 2 (CO) 6 (μ-adt)CH 2 C 6 H 5 ] catalyst, MPA-CdTe QDs, chitosan and H 2 A. A maximal rate of H 2 evolution was achieved at pH 4.5, whereas significant amounts of H 2 were also observed at either lower or higher pH value. This pH-dependent effect should be related to the solubility of chitosan, the stability of MPA-CdTe QDs and the equilibrium of H 2 A=H + +HA − . At a higher pH value, the lack of protonatable amine groups at C-2 position of the glucosamine residue [54] decreases the solubility of chitosan and thus lowers the ability of chitosan to function as an environmental confinement. On the other hand, the protons in the solution with lower pH would suppress the equilibrium to generate enough sacrificial electron donor of HA − for H 2 evolution [45] , and at the same time the MPA ligands would dissociate from the surface of CdTe QDs at a pH value of the solution lower than 4.0, resulting in precipitation and defects that could capture the excited electrons on the surface of the MPA-CdTe species [55] , [56] . Considering all above experimental trials, we carried out the reaction under the optimized condition, that is, 10 ml methanol/water solution (1:3 v-v) containing [Fe 2 (CO) 6 (μ-adt)CH 2 C 6 H 5 ] catalyst (1.00 × 10 −6 mol l −1 ), MPA-CdTe QDs (1.71 × 10 −6 mol l −1 ), H 2 A (0.10 mol l −1 ) and chitosan (1.0 g l −1 ) at pH 4.5. More than 1.04±0.04 ml of H 2 was produced during 10 h of irradiation with visible light ( λ =410 nm) ( Supplementary Fig. S4 ). Even more amounts of H 2 in a total of 11.83±0.39 ml were obtained when the concentration of H 2 A was further increased to 0.20 mol l −1 ( Supplementary Fig. S6 ). This result means that more than (5.28±0.17) × 10 4 equivalents of H 2 per [Fe 2 (CO) 6 (μ-adt)CH 2 C 6 H 5 ] catalyst are generated over 60 h of irradiation ( Fig. 2d ), with an initial TOF of 1.40±0.22 H 2 per catalyst per second in the first 2 h ( Supplementary Fig. S7 ). The catalytic activity is improved 4.16 × 10 3 folds that of the same system without chitosan. Interaction of catalytic components with chitosan The enhanced durability and efficiency is possibly due to the strong interaction and close contact between the MPA-CdTe QDs, [Fe 2 (CO) 6 (μ-adt)CH 2 C 6 H 5 ] catalyst and H 2 A in the chitosan-confined environment ( Fig. 1 ). The encapsulation of the MPA-CdTe QDs by chitosan was well evidenced by high-resolution transmission electron microscopy. The high-resolution transmission electron microscopy images of the MPA-CdTe QDs reveal that chitosan associates with the MPA-CdTe QDs to form self-assemblies on a large scale, and their average size is in the range of 50~200 nm ( Fig. 3 ). Even after 10 h of irradiation, the shape and composition of the self-assemblies with well-crystallized lattices of MPA-CdTe QDs for H 2 evolution remained unchanged. This finding is different from that observed in the reaction system without chitosan ( Supplementary Fig. S8 ). Although no obvious spectral change could be detected in the UV–vis absorption spectra of chitosan and MPA-CdTe QDs as well as their mixture ( Supplementary Fig. S9 ), the photoluminescent intensity of the MPA-CdTe QDs increased and blue-shifted greatly with the introduction of chitosan ( Fig. 4a ), and simultaneously the photoluminescent lifetime of the MPA-CdTe QDs enhanced from 10.9 to 18.3 ns when the concentration of chitosan was varied from 0 to 1.0 g l −1 at pH 4.5 ( Fig. 4b ). It is known that the photoluminescence of QDs is very sensitive to a pH value of solution [55] . When the pH value of an aqueous solution of the MPA-CdTe was adjusted to 4.5, the maximal photoluminescence was found to shift to lower energy at 575 nm accompanying with decreases in the photoluminescent intensity and lifetime ( Table 1 ). The observations are due to the aggregation of the MPA-CdTe QDs to form larger ones [55] , [56] . The blue-shift from 575 to 557 nm in the current study suggests that chitosan stabilizes the CdTe QDs and prevents them from forming larger aggregators. More strikingly, the photoluminescence quantum yield of the MPA-CdTe QDs increased from 5.1% to 38.3% when chitosan was presented in the solution of methanol/water (1:3, v-v) at pH 4.5. The photoluminescent enhancement in intensity, lifetime and quantum yield indicates that chitosan wraps the MPA-CdTe QDs by coordination to cadmium ions of CdTe QDs, and thus suppresses, to some extent, the non-radiative decay of MPA-CdTe QDs. The similar effect was also observed by Yang and Gao et al. [57] with the addition of poly(acrylic acid) into the aqueous solution of CdTe QDs. 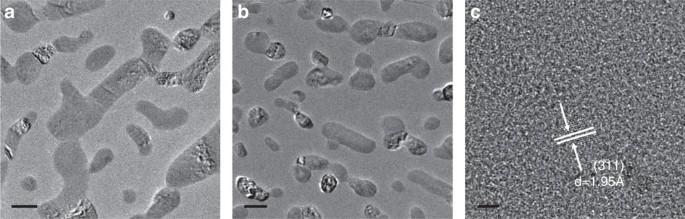Figure 3: Interaction of MPA-CdTe QDs with chitosan. High-resolution transmission electron microscopy images of MPA-CdTe QDs and chitosan in the reaction system before irradiation (a) (bar scale, 200 nm) and after irradiation for 10 h (b) (bar scale, 200 nm). The MPA-CdTe QDs inside chitosan after irradiation for 10 h (c) (bar scale, 2 nm). Figure 3: Interaction of MPA-CdTe QDs with chitosan. High-resolution transmission electron microscopy images of MPA-CdTe QDs and chitosan in the reaction system before irradiation ( a ) (bar scale, 200 nm) and after irradiation for 10 h ( b ) (bar scale, 200 nm). The MPA-CdTe QDs inside chitosan after irradiation for 10 h ( c ) (bar scale, 2 nm). 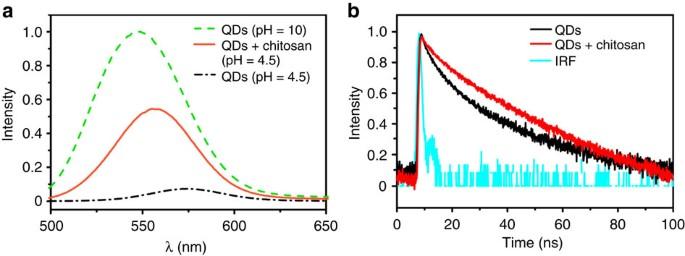Figure 4: Photoluminescence properties of MPA-CdTe QDs with chitosan. (a) Photoluminescence spectra of MPA-CdTe QDs (0.86 × 10−6mol l−1) at pH 10 and pH 4.5, and the photoluminescence of MPA-CdTe in the presence of chitosan at pH 4.5, in methanol/water (1:3 v-v). (b) Photoluminescence lifetime of MPA-CdTe QDs in the absence and presence of chitosan (1.0 g l−1) at pH 4.5. The signal of IRF (blue) is the response of the instrument. Full size image Figure 4: Photoluminescence properties of MPA-CdTe QDs with chitosan. ( a ) Photoluminescence spectra of MPA-CdTe QDs (0.86 × 10 −6 mol l −1 ) at pH 10 and pH 4.5, and the photoluminescence of MPA-CdTe in the presence of chitosan at pH 4.5, in methanol/water (1:3 v-v). ( b ) Photoluminescence lifetime of MPA-CdTe QDs in the absence and presence of chitosan (1.0 g l −1 ) at pH 4.5. The signal of IRF (blue) is the response of the instrument. Full size image Table 1 Spectroscopic and electrochemical properties of the systems for H 2 evolution. Full size table The interaction of [Fe 2 (CO) 6 (μ-adt)CH 2 C 6 H 5 ] catalyst with chitosan was carefully examined and is shown in Fig. 5 . No absorbance could be detected from [Fe 2 (CO) 6 (μ-adt)CH 2 C 6 H 5 ] catalyst in pure water but with continuous sonication of insoluble [Fe 2 (CO) 6 (μ-adt)CH 2 C 6 H 5 ] catalyst and a chitosan (1.0 g l −1 ) solution in methanol/water (1:3, v-v) at pH 4.5 its solubility and absorbance were remarkably enhanced with the formation of a coloured solution. Alternatively, progressive addition of [Fe 2 (CO) 6 (μ-adt)CH 2 C 6 H 5 ] catalyst in dichloromethane into a solution of chitosan (1.0 g l −1 ) in methanol/water (1:3, v-v) at pH 4.5 resulted in an increase of absorption band at 336 nm remarkably. As compared with the same system without chitosan in methanol/water (1:3, v-v) at pH 4.5 ( Supplementary Fig. S10 ), the increment of the absorbance at 336 nm is much greater. The results indicate that water-insoluble [Fe 2 (CO) 6 (μ-adt)CH 2 C 6 H 5 ] catalyst is incorporated into the chitosan solution. The absorbance at 336 nm obeys the Beer’s law showing that [Fe 2 (CO) 6 (μ-adt)CH 2 C 6 H 5 ] catalyst is well dispersed in the chitosan solution at pH 4.5. Decreasing the pH of the solution has no noticeable influence on the absorption spectra, suggesting that [Fe 2 (CO) 6 (μ-adt)CH 2 C 6 H 5 ] catalyst does not react with protons under the experimental condition. 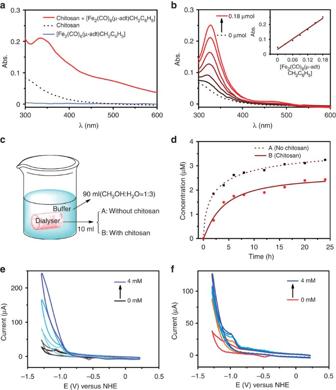Figure 5: Interaction of [Fe2(CO)6(μ-adt)CH2C6H5] catalyst with chitosan. (a) The absorption spectra of [Fe2(CO)6(μ-adt)CH2C6H5] catalyst (3.00 × 10−7mol) in water at pH 4.5, an chitosan solution (1.0 g l−1) in methanol/water (1:3, v-v) at pH 4.5 and [Fe2(CO)6(μ-adt)CH2C6H5] catalyst (3.00 × 10−7mol) with continuous sonication of the chitosan solution (1.0 g l−1) in methanol/water (1:3, v-v) at pH 4.5. (b) The absorption spectra of chitosan (1.0 g l−1) with progressive addition of [Fe2(CO)6(μ-adt)CH2C6H5] (1.00 × 10−3mol l−1in CH2Cl2) in methanol/water (1:3, v-v) at pH 4.5; inset: the absorbance at 336 nm as a function of amounts of [Fe2(CO)6(μ-adt)CH2C6H5] catalyst. (c) The schematic representation of dialysis experiment: the 10 ml solution inside the dialyser containing [Fe2(CO)6(μ-adt)CH2C6H5] catalyst (1.00 × 10−4mol l−1) in the absence (A) and presence (B) of chitosan (1.0 g l−1) in methanol/water (1:3, v-v) at pH 4.5; the solution outside the dialyser containing 90 ml of methanol/water (1:3, v-v) at pH 4.5. (d) The time course of the concentration changes of [Fe2(CO)6(μ-adt)CH2C6H5] catalyst outside the solution of dialysis bag A and dialysis bag B, respectively, which was read from UV–vis absorption spectra. (e) Cyclic voltammograms of [Fe2(CO)6(μ-adt)CH2C6H5] catalyst (2.0 × 10−4mol l−1) in the absence and presence of HOAc in methanol/water (1:1, v-v). (f) Cyclic voltammograms of [Fe2(CO)6(μ-adt)CH2C6H5] catalyst (2.0 × 10−4mol l−1) in the absence and presence of HOAc in methanol/water (1:1, v-v) with chitosan (1.0 g l−1). Figure 5: Interaction of [Fe 2 (CO) 6 (μ-adt)CH 2 C 6 H 5 ] catalyst with chitosan. ( a ) The absorption spectra of [Fe 2 (CO) 6 (μ-adt)CH 2 C 6 H 5 ] catalyst (3.00 × 10 −7 mol) in water at pH 4.5, an chitosan solution (1.0 g l −1 ) in methanol/water (1:3, v-v) at pH 4.5 and [Fe 2 (CO) 6 (μ-adt)CH 2 C 6 H 5 ] catalyst (3.00 × 10 −7 mol) with continuous sonication of the chitosan solution (1.0 g l −1 ) in methanol/water (1:3, v-v) at pH 4.5. ( b ) The absorption spectra of chitosan (1.0 g l −1 ) with progressive addition of [Fe 2 (CO) 6 (μ-adt)CH 2 C 6 H 5 ] (1.00 × 10 −3 mol l −1 in CH 2 Cl 2 ) in methanol/water (1:3, v-v) at pH 4.5; inset: the absorbance at 336 nm as a function of amounts of [Fe 2 (CO) 6 (μ-adt)CH 2 C 6 H 5 ] catalyst. ( c ) The schematic representation of dialysis experiment: the 10 ml solution inside the dialyser containing [Fe 2 (CO) 6 (μ-adt)CH 2 C 6 H 5 ] catalyst (1.00 × 10 −4 mol l −1 ) in the absence (A) and presence (B) of chitosan (1.0 g l −1 ) in methanol/water (1:3, v-v) at pH 4.5; the solution outside the dialyser containing 90 ml of methanol/water (1:3, v-v) at pH 4.5. ( d ) The time course of the concentration changes of [Fe 2 (CO) 6 (μ-adt)CH 2 C 6 H 5 ] catalyst outside the solution of dialysis bag A and dialysis bag B, respectively, which was read from UV–vis absorption spectra. ( e ) Cyclic voltammograms of [Fe 2 (CO) 6 (μ-adt)CH 2 C 6 H 5 ] catalyst (2.0 × 10 −4 mol l −1 ) in the absence and presence of HOAc in methanol/water (1:1, v-v). ( f ) Cyclic voltammograms of [Fe 2 (CO) 6 (μ-adt)CH 2 C 6 H 5 ] catalyst (2.0 × 10 −4 mol l −1 ) in the absence and presence of HOAc in methanol/water (1:1, v-v) with chitosan (1.0 g l −1 ). Full size image The interaction of [Fe 2 (CO) 6 (μ-adt)CH 2 C 6 H 5 ] catalyst and chitosan was further confirmed by dialysis experiments. As depicted in the schematic representation of Fig. 5 , 1.00 × 10 −4 mol l −1 of [Fe 2 (CO) 6 (μ-adt)CH 2 C 6 H 5 ] catalyst was put into dialysis bag A, and the same amount of [Fe 2 (CO) 6 (μ-adt)CH 2 C 6 H 5 ] catalyst together with 1.0 g l −1 of chitosan were in dialysis bag B, respectively. Along with the time, the diffusion rate of the catalyst to the outside solution from dialysis bag B was noted much slower than that from dialysis bag A, and thus leading to the concentration change of the catalyst from dialysis bag B smaller than that from dialysis bag A. These results imply the intimate interaction of chitosan and [Fe 2 (CO) 6 (μ-adt)CH 2 C 6 H 5 ] catalyst. The direct evidence on the interaction comes from electrochemical studies under nitrogen atmosphere. Note that the reduction potential of [Fe 2 (CO) 6 (μ-adt)CH 2 C 6 H 5 ] positively shifts from −1.36 V versus NHE in acetonitrile to −1.10 V versus NHE in methanol/water (1:1, v-v) at pH 4.5 ( Supplementary Fig. S11 ), which is attributed to the reduction of Fe I Fe I to Fe I Fe 0 of [Fe 2 (CO) 6 (μ-adt)CH 2 C 6 H 5 ] catalyst [27] , [28] , [29] . Although the reduction potential of [Fe 2 (CO) 6 (μ-adt)CH 2 C 6 H 5 ] remained unchanged with the addition of chitosan at pH 4.5 ( Table 1 ), the cyclic voltammogram of a solution with or without chitosan, containing the same amounts of [Fe 2 (CO) 6 (μ-adt)CH 2 C 6 H 5 ] catalyst, displayed different electrochemical responses on progressive addition of acetic acid (HOAc). Given in Fig. 5 is the cyclic voltammetry of [Fe 2 (CO) 6 (μ-adt)CH 2 C 6 H 5 ] catalyst in the absence and presence of HOAc. The current intensity of the reduction peak increases with the acid concentration, the characteristic of proton reduction [10] , [11] , [12] . On reversing the scan following the reductions at −1.26 V versus NHE, a reproducible curve-crossing was clearly observed for [Fe 2 (CO) 6 (μ-adt)CH 2 C 6 H 5 ] catalyst resulting in the buildup of current response at −1.00 V versus NHE. The peak current at −1.00 V is proportional to the square root of the scan rate ( Supplementary Fig. S12 ), suggesting that the electrochemical processes are diffusion-controlled and excluding the possibility of the curve-crossing event arising from electrode deposition. Moreover, the current height of the −1.00 V events increases with increasing acid concentrations. Its dependence on both potential scan rate and acid concentration reveals that a larger fraction of the starting material is regenerated at reaction times that correspond to potentials positive of the curve-crossing. Following from the electrochemical studies of a mimic of the diiron subunit of [FeFe]-H 2 ase by Darensbourg and co-workers [28] , we suppose that the curve-crossing electrochemical responses are an integral property of the electroactive (−1.10 V) species, presumed to be the Fe I Fe I to Fe I Fe 0 reduction, for which a rapid chemical reaction, that is, protonation of the Fe I Fe 0 species produces the increased current at more negative potential. The presence of a more easily reproducible product or intermediate as seen in the reverse electrochemical scan suggests that a subsequent slow chemical reaction produces an intermediate of sufficient stability to build up in solution and migrate back to the electrode for reduction at a more positive potential. Evidently, the system with chitosan yielded much more intermediate species at −1.00 V than that working in the absence of chitosan under the same concentration of [Fe 2 (CO) 6 (μ-adt)CH 2 C 6 H 5 ] catalyst, indicative of greater sensitivity and stability of the reduced species to acid concentration in the presence of chitosan. In view of the sensitivity of the system to the pH value of solution, all of the interaction studies were carried out at pH 4.5 to agree with the optimized condition. In the presence of chitosan, the absorption spectrum of the MPA-CdTe QDs and [Fe 2 (CO) 6 (μ-adt)CH 2 C 6 H 5 ] catalyst was the superposition of the MPA-CdTe QDs, chitosan and [Fe 2 (CO) 6 (μ-adt)CH 2 C 6 H 5 ] ( Supplementary Fig. S9 ), but the photoluminescence of MPA-CdTe QDs was quenched by [Fe 2 (CO) 6 (μ-adt)CH 2 C 6 H 5 ] dramatically. As shown in Fig. 6 , excitation of the characteristic absorption of MPA-CdTe QDs resulted in a maximal photoluminescence at 575 nm in methanol/water (1:3, v-v) solution, which was quenched by [Fe 2 (CO) 6 (μ-adt)CH 2 C 6 H 5 ] with a rate constant of (9.95±0.67) × 10 3 l mol −1 ( Table 1 , Supplementary Fig. S13 ). When 1.0 g l −1 of chitosan was presented in the solution, the photoluminescent maximum blue-shifted to 557 nm and the quenching rate constant increased to (2.26±0.02) × 10 4 l mol −1 ( Table 1 , Supplementary Fig. S13 ). Clearly, the interaction between the MPA-CdTe QDs and [Fe 2 (CO) 6 (μ-adt)CH 2 C 6 H 5 ] catalyst is stronger in the self-assembled chitosan system than that in free solution. 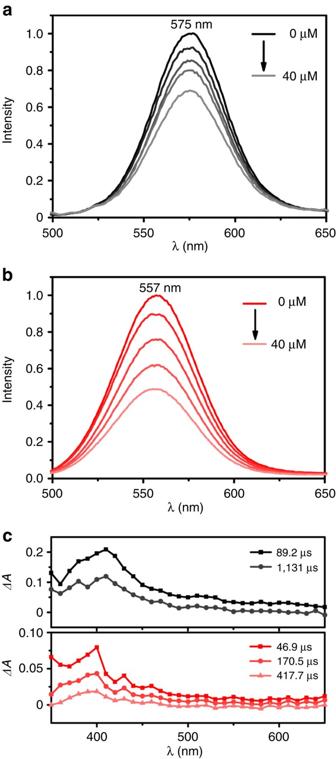Figure 6: Interaction of MPA-CdTe QDs and [Fe2(CO)6(μ-adt)CH2C6H5] with chitosan. (a) Photoluminescence quenching of MPA-CdTe QDs (0.86 × 10−6mol l−1) with progressive addition of [Fe2(CO)6(μ-adt)CH2C6H5] catalyst in the absence of chitosan. (b) Photoluminescence quenching of MPA-CdTe QDs (0.86 × 10−6mol l−1) with progressive addition of [Fe2(CO)6(μ-adt)CH2C6H5] catalyst in the presence of chitosan. (c) Transient absorption spectra of MPA-CdTe QDs (0.86 × 10−6mol l−1) and [Fe2(CO)6(μ-adt)CH2C6H5] catalyst (5.00 × 10−5mol l−1) in the absence (top) and presence (bottom) of chitosan in methanol/water (1:3 v-v) at pH 4.5. Figure 6: Interaction of MPA-CdTe QDs and [Fe 2 (CO) 6 (μ-adt)CH 2 C 6 H 5 ] with chitosan. ( a ) Photoluminescence quenching of MPA-CdTe QDs (0.86 × 10 −6 mol l −1 ) with progressive addition of [Fe 2 (CO) 6 (μ-adt)CH 2 C 6 H 5 ] catalyst in the absence of chitosan. ( b ) Photoluminescence quenching of MPA-CdTe QDs (0.86 × 10 −6 mol l −1 ) with progressive addition of [Fe 2 (CO) 6 (μ-adt)CH 2 C 6 H 5 ] catalyst in the presence of chitosan. ( c ) Transient absorption spectra of MPA-CdTe QDs (0.86 × 10 −6 mol l −1 ) and [Fe 2 (CO) 6 (μ-adt)CH 2 C 6 H 5 ] catalyst (5.00 × 10 −5 mol l −1 ) in the absence (top) and presence (bottom) of chitosan in methanol/water (1:3 v-v) at pH 4.5. Full size image As the spectral overlap of absorption of [Fe 2 (CO) 6 (μ-adt)CH 2 C 6 H 5 ] catalyst and photoluminescence of MPA-CdTe QDs is rather small, the energy transfer from the excited MPA-CdTe QDs to [Fe 2 (CO) 6 (μ-adt)CH 2 C 6 H 5 ] catalyst would be negligible. Electron transfer from the excited MPA-CdTe QDs to [Fe 2 (CO) 6 (μ-adt)CH 2 C 6 H 5 ] catalyst is therefore responsible for the photoluminescence quenching of the MPA-CdTe QDs. Combining electrochemical and spectroscopic studies ( Table 1 ), we estimated the free-energy change of electron transfer reaction from the excited MPA-CdTe QDs to [Fe 2 (CO) 6 (μ-adt)CH 2 C 6 H 5 ] catalyst. According to the valence-band energy level ( E vb ) of MPA-CdTe QDs, which is 0.09 V (all potentials discussed here are versus NHE) [58] and the reduction potential ( E red ) of [Fe 2 (CO) 6 (μ-adt)CH 2 C 6 H 5 ] catalyst determined as −1.10 V in methanol/water (1:1, v-v) at pH 4.5 ( Table 1 ), the excited-state energy ( E 00 ) of MPA-CdTe QDs being 2.23 eV in the presence of chitosan and 2.16 eV in the absence of chitosan at pH 4.5 ( Table 1 ), respectively, the free-energy change (Δ G 0 ) of the electron transfer reaction was thus calculated to be −1.04 eV in the presence of chitosan and −0.97 eV in the absence of chitosan at pH 4.5 ( Table 1 , Supplementary Fig. S14 ). This means that the electron transfer from the excited MPA-CdTe QDs to [Fe 2 (CO) 6 (μ-adt)CH 2 C 6 H 5 ] catalyst in this designed system is more exothermic. Flash photolysis study provides direct evidence on the photoinduced electron transfer process at room temperature. On laser excitation of the MPA-CdTe QDs using 355 nm light, no characteristic absorption signal was observed from ultraviolet to visible region under the time scale of 2.0 μs ( Supplementary Fig. S15 ). When [Fe 2 (CO) 6 (μ-adt)CH 2 C 6 H 5 ] catalyst was added into the MPA-CdTe QDs solution containing 1.0 g l −1 of chitosan, a new set of absorption bands emerged immediately ( Fig. 6c ). The generated new absorption is similar to that of [Fe 2 (CO) 6 (μ-adt)CH 2 C 6 H 5 ] catalyst under reduction potential at −1.16 V versus NHE in methanol/water (1:1, v-v) at pH 4.5 ( Supplementary Fig. S15 ), in line with the Fe I Fe 0 species reported by Pickett and co-workers [29] using the same approach. Therefore, the absorption ~410 nm is attributed to the Fe I Fe 0 species generated by electron transfer from the excited MPA-CdTe QDs to [Fe 2 (CO) 6 (μ-adt)CH 2 C 6 H 5 ]. As that of the MPA-CdTe QDs after delivering an electron to [Fe 2 (CO) 6 (μ-adt)CH 2 C 6 H 5 ] catalyst might show absorptions in this region though no signal was detected on laser excitation of MPA-CdTe QDs itself in methanol/water (1:3, v-v) at pH 4.5, we proposed that the transient signals at ~410 nm may result from the spectral overlap of both Fe I Fe 0 species and that of the CdTe QDs after electron transfer. The active Fe I Fe 0 species from [Fe 2 (CO) 6 (μ-adt)CH 2 C 6 H 5 ] catalyst can further react with protons to experience catalytic cycle for H 2 evolution. The formed hole remaining in the MPA-CdTe species after electron transfer, on the other hand, is subsequently regenerated by electron transfer from the sacrificial electron donor. It is known that the redox potential of H 2 A (−0.14 V at pH 4.5) [59] is sufficiently negative to reduce the holes photogenerated in MPA-CdTe species [25] , [45] , but it is too positive to directly reduce the [FeFe]-H 2 ase catalyst ( Supplementary Fig. S14 ). Therefore, the holes left in CdTe QDs are consumed by the sacrificial electron donor H 2 A. To examine the possibility of chitosan to function as another electron donor, we did the experiment for H 2 evolution in the absence of H 2 A at pH 4.5 ( Supplementary Fig. S2 ). But no H 2 could be detected in the system, indicative that the functionality of chitosan to serve as a sacrificial electron donor would be negligible. In this case, one may speculate that when the MPA-CdTe QDs is excited by visible light, the electron transfer from the conduction band of MPA-CdTe QDs to [Fe 2 (CO) 6 (μ-adt)CH 2 C 6 H 5 ] catalyst takes place giving rise to the reduced [Fe 2 (CO) 6 (μ-adt)CH 2 C 6 H 5 ]. At the same time, the holes remaining in the valence band of MPA-CdTe QDs after electron transfer are regenerated by electron transfer from the sacrificial ascorbic acid H 2 A to complete the photocatalytic cycle ( Supplementary Fig. S14 ). As compared with those reported in the literature [34] , [35] , [36] , [37] , [38] , [39] , [40] , [41] , [42] , [43] , [44] , [45] , [46] , [47] , [48] , [49] , [50] , [51] , the durability and activity of the present system are greatly increased; possibly as a result of the stabilization of the components by chitosan confinement leading to consecutive multi-step electron transfer in equilibrium. The importance of the stabilization was also analysed by exchanging chitosan for relatively small and loose aggregates, anionic SDS (0.166 mol l −1 ) and cationic CTAB (0.055 mol l −1 , cetyl trimethyl ammonium bromide) micelles [37] . For systematic comparison, the photocatalytic H 2 evolution experiment was carried out from the same reaction system, containing MPA-CdTe QDs, [Fe 2 (CO) 6 (μ-adt)CH 2 C 6 H 5 ] catalyst and H 2 A, in SDS and CTAB micelles, respectively. The TON is only 37.6±3.2 and 36.0±4.4 for the SDS and CTAB system, respectively, even after irradiation for 10 h ( Supplementary Fig. S16 ). Notably, these solutions were quickly changed from orange to brownish red with the formation of brown precipitates on irradiation, whereas the chitosan-involved system was clear even after 40 h irradiation. The results demonstrate that the chitosan-confined H 2 -evolving system has more advantage over the micellar systems. The significant content of hydroxyl group and protonated amines of polycationic chitosan has shown affinity towards the negative MPA-CdTe QDs, [Fe 2 (CO) 6 (μ-adt)CH 2 C 6 H 5 ] catalyst and H 2 A, which improves the electron transfer processes from the MPA-CdTe QDs to [Fe 2 (CO) 6 (μ-adt)CH 2 C 6 H 5 ], as well as H 2 A to the holes of MPA-CdTe QDs after electron transfer (see above). Because two electrons are required to produce each molecule of H 2 , the stabilization of the MPA-CdTe QDs, [Fe 2 (CO) 6 (μ-adt)CH 2 C 6 H 5 ] catalyst and catalytic intermediate and the consecutive multi-step electron transfer in equilibrium are believed to be responsible for the regeneration of the MPA-CdTe species and [Fe 2 (CO) 6 (μ-adt)CH 2 C 6 H 5 ] catalyst to improve the efficiency of H 2 evolution in the chitosan-confined system. Unlike most state-of-the-art approaches, the system does not rely on further structure modification of butterfly [Fe 2 S 2 ] subunit but on the addition of natural polysaccharide chitosan. The catalytic performance has been improved from 12.7±1.3 to (5.28±0.17) × 10 4 turnover numbers under the same condition, which increases 4.16 × 10 3 folds as compared with the same system without chitosan. These results imply that the environmental protein surrounding catalytic centre might cause the significant activity difference between the diiron subsite of natural [FeFe]-H 2 ase and its synthetic mimics. The crucial role of chitosan suggests that to create active H 2 evolution systems based on artificial [FeFe]-H 2 ases, one would need to mimic not only the structure of active centre but also the biological environment surrounding [Fe 2 S 2 ] subunit. The present artificial system using chitosan-confined environment is reminiscent of the [Fe 2 S 2 ] subcluster of natural [FeFe]-H 2 ase buried in heterogeneous protein matrix, and demonstrates that artificial [FeFe]-H 2 ases are promising alternatives for use in a future sustainable H 2 economy. Chemicals and synthesis All reagents were weighed and handled in air, and backfilled under an inert atmosphere of argon at room temperature. Chitosan (low molecular weight, 20–300 cP, 1 wt. % in 1% acetic acid (25 °C, Brookfield (lit. )), L-ascorbic acid (H 2 A, 99%), MPA (99%) and CdCl 2 ·2.5H 2 O (99%) were purchased from Sigma-Aldrich. Benzylamine (97%) and paraformaldehyde (97%) were purchased from Alfa-Aesar. All commercial chemicals are used without further purification unless otherwise noted. The ultrapure water with 18.2 MΩ cm (Mettler Toledo, FE20) was used throughout the experiment. The [Fe 2 (CO) 6 (μ-adt)CH 2 C 6 H 5 ] catalyst was synthesized by the reaction of benzylamine, aldacide, thionylchloride and the lithium salt of diiron hexacarbonyldisulphide as that repoted in the previous work [27] , [37] . The aqueous colloidal MPA-CdTe QDs solution was prepared using the reaction between Cd 2+ and NaHTe solution according to the literature [45] . Cd 2+ precursor solutions were prepared by mixing the solutions of CdCl 2 ·2.5H 2 O and stabilizer (MPA) followed by pH adjustment to 10 with 1 mol l −1 NaOH and degassed by bubbling nitrogen for 30 min. Then a fresh NaHTe was added under anaerobic condition in a typical molar ratio of Cd:MPA:Te as 1:1.2:0.2. The resulting solution was then heated to 99–100 °C after bubbling nitrogen for another 30 min and refluxed in different reaction time to control the size of MPA-CdTe QDs. Aliquots of the reaction solution were taken out at regular intervals for UV–vis absorption and photoluminescence characterization. Photocatalytic H 2 evolution A typical procedure for H 2 production is as follows. Chitosan (10 mg) and H 2 A (2.00 × 10 −3 mol) were dissolved in 3.50 ml water and diluted with the 2.49 ml methanol with vigorous stirring. The excess acid was then neutralized by adding NaOH (5.0 mol l −1 ) solution and adjusted the solution to weakly acidic (pH 4~5). Then, 4.00 ml of aqueous MPA-CdTe QDs solution (1.71 × 10 −6 mol l −1 ), 10.0 μl of methanol solution containing [Fe 2 (CO) 6 (μ-adt)CH 2 C 6 H 5 ] catalyst (1.00 × 10 −3 mol l −1 ) were added to the above solution (total volume became 10 ml) with stirring. The pH value of the mixed solution was further adjusted to 4.5 by aqueous 1.0 mol l −1 HCl and determined by a pH meter. The sample was degassed by bubbling nitrogen for 30 min. Then 1,000 μl of CH 4 was injected as the internal standard for quantitative GC analysis. The sample was irradiated by light-emitting diodes ( λ =410 nm). The generated photoproduct of H 2 was characterized by GC analysis (Tianmei 7890-II) using nitrogen as the carrier gas with a molecular sieve column (5 Å) and a thermal conductivity detector. Then 400 μl of mixed gas was extracted from the sample tube and injected into the GC immediately. The response factor for H 2 /CH 4 was about 5.10 under the experimental condition, which was established by calibration with known amounts of H 2 and CH 4 and determined before and after a series of measurements. The desired concentration of reaction system was achieved by dissolving different amount of chitosan, H 2 A, the MPA-CdTe QDs and [Fe 2 (CO) 6 (μ-adt)CH 2 C 6 H 5 ] catalyst into 10 ml of the mixed aqueous solution. Absorption and photoluminescence measurements UV–vis spectra were measured on a Shimadzu UV-1601PC spectrophotometer in a quartz cell with an optical path length of 1 cm. The interaction of [Fe 2 (CO) 6 (μ-adt)CH 2 C 6 H 5 ] catalyst (0.30 × 10 −6 mol, solid) and chitosan (1.0 g l −1 , in methanol/water (1:3, v-v)) was sonicated for 15 min before measurement. Photoluminescence was recorded on a Hitachi F-4500 spectrofluorimeter at room temperature. Photoluminescence lifetime was measured on the Edinburgh FLSP920 with excitation at 405 nm. The photoluminescence quenching experiment was performed by progressive addition of [Fe 2 (CO) 6 (μ-adt)CH 2 C 6 H 5 ] catalyst (1.0 × 10 −3 mol l −1 , in methanol) into the solution at pH 4.5. The volume of [Fe 2 (CO) 6 (μ-adt)CH 2 C 6 H 5 ] catalyst added to the system is so small that the volume change is ignored in the determination of the concentration. Dialysis experiments The dialyser bags (purchased from Biotopped, molecular weight cutoff 3,500) were pretreated with hot water and kept in deionized water before use. Mixed solution (10 ml) containing [Fe 2 (CO) 6 (μ-adt)CH 2 C 6 H 5 ] and chitosan was loaded into the dialyser bag. Then, the seal-off dialyser bag was soaked in 90 ml solution of methanol/water (1:3, v-v) in the dark. UV–vis absorption spectrometer was employed to examine the concentration of [Fe 2 (CO) 6 (μ-adt)CH 2 C 6 H 5 ] outside dialysis bag. Electrochemical and spectroelectrochemical measurements A three-electrode system was used for the measurement and bulk electrolysis, with a 3-mm glass carbon working electrode, a platinum wire counter electrode and a non-aqueous Ag/AgNO 3 reference electrode for organic solution or a saturated calomel electrode (SCE) reference electrode for aqueous solution. The working electrode was polished with a 0.05 μm alumina paste and sonicated for 15 min before use. The electrolyte solution (0.1 mol l −1 of n -Bu 4 NPF 6 in acetonitrile for organic solution, 0.1 mol l −1 of Na 2 SO 4 for methanol/water (1:1 v-v) solution) was purged with argon for 30 min before measurement. Spectroelectrochemical experiment was performed in a quartz cell with an optical path length of 1 cm. Indium tin oxide glass was used as a working electrode and a platinum wire electrode and a SCE reference electrode were served as the counter and reference electrodes, respectively. The electrolyte solution was purged with argon for 30 min before the absorption spectra were recorded on a Shimadzu UV-1601PC spectrometer. Spectroelectrochemical absorption spectrum was recorded along with time of electrochemical reduction of [Fe 2 (CO) 6 (μ-adt)CH 2 C 6 H 5 ] catalyst at −1.4 V relative to SCE (−1.16 V versus NHE) in methanol/water (1:1, v-v), the baseline of which refers to the absorption of [Fe 2 (CO) 6 (μ-adt)CH 2 C 6 H 5 ] catalyst before reduction under the voltage. Flash photolysis The transient absorption spectroscopy was recorded on Edinburgh LP 920 at room temperature. A mixture of methanol/water (1:3 v-v) solution was degassed with nitrogen for 30 min before measurement. Excitation was provided using Nd:YAG laser (third harmonic, 10 ns) at 355 nm and the detector was a xenon lamp on the Edinburgh LP 920 apparatus. How to cite this article: Jian, J.-X. et al. Chitosan confinement enhances hydrogen photogeneration from a mimic of the diiron subsite of [FeFe]-hydrogenase. Nat. Commun. 4:2695 doi: 10.1038/ncomms3695 (2013).